Sprite streamer initiation from natural mesospheric structures Sprites are large, luminous electrical discharges in the upper atmosphere caused by intense cloud-to-ground lightning flashes, manifesting an impulsive coupling mechanism between lower and upper atmospheric regions. Their dynamics are governed by filamentary streamer discharges whose propagation properties have been well studied by past work. However, how they are initiated is still under active debate. It has recently been concluded that ionospheric/mesospheric inhomogeneities are required for their initiation, but it is an open question as to what the sources of those inhomogeneities are. Here we present numerical simulation results to demonstrate that naturally-existing, small-scale mesospheric structures such as those created by gravity waves via instability and breaking are viable sources. The proposed theory is supported by a recent, unique high-speed observation from aircraft flying at 14-km altitude. The theory naturally explains many aspects of observed sprite streamer initiation and has important implications for future observational work. Intense cloud-to-ground (CG) lightning flashes are capable of generating a brief, strong quasi-electrostatic (QE) field in the mesosphere/lower ionosphere to trigger electrical discharges known as sprites [1] , [2] , [3] , [4] . The observation of sprites was first reported in scientific literature in the early 1990s [5] . Subsequent work indicated that they appear above thunderstorms within a few to hundreds of milliseconds from the parent lightning and may span an altitude range of 40–90 km (refs 6 , 7 ). The luminosity of a sprite persists only for a few to tens of milliseconds, but its electrical and chemical effects last much longer [7] . It has been found that filamentary streamer discharges are the building blocks of sprites [8] , [9] , [10] . A streamer is a highly nonlinear ionization wave that can propagate self-consistently in an electric field below the air breakdown threshold field by carrying a strongly enhanced field region at its wave front. The propagation characteristics of a single sprite streamer, such as acceleration, expansion and brightening, are relatively well understood [10] , [11] , [12] , [13] , [14] , [15] , [16] , [17] , [18] . However, how sprite streamers are initiated, a critical question to understand the responses of the upper atmosphere to sudden, strong QE field impacts, is still under active debate [14] , [19] , [20] , [21] , [22] , [23] , [24] , [25] , [26] . In particular, recent observation-based studies indicate that sprites can be initiated even if the lightning electric field is only about a few tenths of the breakdown threshold field E k [27] , [28] . Those studies also show that about half of the observed sprites appear after a more than 10 ms delay from the causative CGs [27] , and they are initiated around 70-km altitude, lower than that of prompt sprites [27] , [28] , [29] . The long-continuing current of the parent lightning can maintain a moderate electric field at the sprite initiation altitude, and sometimes sprite initiation occurs during a 5–20 ms rise of the current [27] . However, there is no indication of sudden crossing of a certain threshold condition at the moment of sprite initiation. Another important observational finding is that some streamers of prompt sprites are initiated from visible structures in preceding halos, while the streamers of delayed sprites normally emerge out of the dark background [30] . Halos are relatively homogeneous glows that are also driven by the QE field of CGs. They typically appear within a few milliseconds of the CGs, and are centred on 78–80-km altitude with a horizontal extent of tens of kilometres and a vertical thickness of several kilometres. A recent study [31] reported detection of a mesospheric irregularity with a volume of 3–19 km 3 at 80–85-km altitude that was illuminated by a lightning flash causing a nearby sprite event. The initiation of sprite streamers at sub-breakdown conditions was addressed by a few recent modelling studies [21] , [22] , [25] . It has been found that streamers can be initiated from thin, dense column ionization patches with a plasma density more than three orders of magnitude, higher than the ambient ionospheric electron density [21] , [22] or from hundreds of metre wide spherical patches with a density about two orders of magnitude higher than the ambient value [25] . Modelling studies have also shown that plasma inhomogeneities with a density of two orders of magnitude higher than the ambient are also required for sprite streamer initiation at overbreakdown conditions [19] , [20] , [23] . The candidate sources of the inhomogeneities include the ionospheric effects of thunderstorm/lightning activities, meteor trails and gravity waves [21] , [22] , but no study has unambiguously demonstrated the feasibility of streamer initiation from the inhomogeneities created by any of those processes. A more recent modelling study has rigorously shown that the dynamic aspects of the luminous halo structures leading to streamer initiation can be reproduced by subjecting a dense (10 8 m −3 ) plasma column of 12-km long and 2-km wide that might be created by meteor trails to a typical lightning field [26] . However, the lifetime of electron density is very short ( ∼ 1 s) at 70-km altitude [32] . It is reasonable to expect that meteor trails do not play a major role in the initiation of the long-delayed sprites, because observed sprites are rarely accompanied by meteors. It is possible that some delayed sprite streamers are initiated by the remnants of previous, dim streamers that are not bright enough to be detected by the high-speed imaging system. According to simulations based on electrical engineering circuit models [33] , another possible mechanism to initiate long-delayed sprites is the moderately strong continuing current of the parent CG, which can generate an electric field greater than E k from 55- to 67-km altitude after a more than 20 ms delay. In this paper, we will consider the possibility of initiation of the long-delayed sprite streamers from small-scale mesospheric structures such as those created by gravity waves. It is known that thunderstorms also generate gravity waves with a full range of spatial scales including short-period, small-scale gravity waves with a wavelength of a few tens of kilometres [34] , [35] , [36] , [37] , [38] , [39] , [40] . The generated gravity waves propagate upwards and spread radially outwards. They reach the mesosphere within tens of minutes and extend laterally hundreds of kilometres or more above the convection core of thunderstorms. The small-scale gravity waves have been observed to create band structures with a typical wavelength range of 20–30 km at the airglow layer around 80–100-km altitude. Smaller, ripple-like structures on the order of 5–20 km can then be produced via instability or breaking, and they are often found to superimpose on the band structure. The instability and breaking of the gravity waves can further result in even smaller turbulent structures. The disturbances associated with the gravity waves typically modify neutral density and temperature by a few per cent. However, because the coefficients of the governing basic discharge processes of electrical discharges in the atmosphere are a very sensitive function of the ratio of electric field and neutral density, a few per cent perturbation in neutral density can result in a few tens of per cent change in those coefficients [10] , [41] . Here we present numerical simulation results to show that small-scale mesospheric structures can initiate sprite streamers under the influence of the lightning electric field inferred from measurements. Our focus is to investigate the initiation of the long-delayed sprites, but a short discussion on prompt sprite initiation is also given. The proposed theory is supported by high-speed images of a long-delayed sprite event recently recorded at aircraft altitude. The combined results from the models and observations indicate that the optical intensity ensemble of halos, streamers and sprites spans a much larger dynamic range than that of the current imaging system. Therefore, many small, dim glows caused by lightning likely elude the detection of current imaging instruments. Model formulation The simulations are conducted by using a cylindrically symmetric plasma discharge model that accounts for all the processes important for electrical discharges in the upper atmosphere. A detailed description of the model can be found in the Methods section. The observational finding that long-delayed sprites are initiated at a few tenths of E k [27] , [28] is generally consistent with the results from a recent halo modelling study [41] . This modelling study shows that the front of a typical halo as an ionization wave descends to 70- to 75-km altitude after a few milliseconds, and the peak electric field becomes smaller than E k . At such a field, ionization growth takes place on a timescale of a few to tens of milliseconds, resulting in the formation of a sharp, almost stationary halo front. Now, if mesospheric perturbations with a spatial scale on the order of the halo front thickness are present in the high-field region of the halo, there will be sufficient time for them to grow through field enhancement, electron density increase, further field enhancement and so on. As shown below, this can eventually lead to streamer initiation. To the spatial scale of sprite streamers, the halo front can be approximated as a planar ionization wave front. Its plasma density profile as a function of height z can be described by a hyperbolic tangent, , which models an intermediate stage of the slowly descending halo front by capturing the rapid plasma density change at the front and approximately constant level behind the front [41] . The front is located at z 0 with a thickness of σ z , and the plasma density behind the front is n 0 . Proper boundary conditions (see Methods) are implemented to ensure accurate modelling of the propagation of this wave front in the lightning electric field. According to the halo simulation results [41] , the lightning electric field near 70-km altitude, below the halo front, slowly varies at a fraction of E k , for example, −(0.5–0.6) E k . This allows the characterization of the ambient electric field condition for streamer initiation by setting the bottom boundary of the simulation domain at an altitude near 70 km and specifying a simple temporal variation (for example, constant) for the normal component of the electric field at this boundary. This set-up not only greatly improves the simulation efficiency but also enables a focused investigation of the role of the mesospheric structure in streamer initiation by giving the streamer model a typical, well-defined input imposed by the halo. If not explicitly mentioned in the paper, the normal component of the electric field at this boundary is kept constant at − E 0 × N 70 / N bottom , where N is the neutral density; that is, the value of E 0 is referenced to 70-km altitude. Test runs were performed to validate this model for simulating planar ionization waves, and an example of those simulations is briefly discussed here and is shown in more detail in Supplementary Fig. 1 . 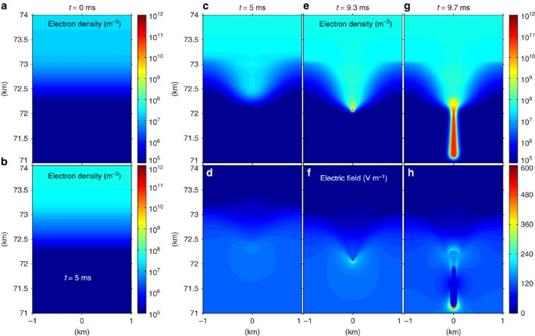Figure 1: Sprite streamer initiation from a halo front deformed by mesospheric structures. (a) Initial electron density distribution. (b) A descending, sharpening halo front that keeps its planar geometry if there is no perturbation. (c–h) A growing mesospheric structure near the halo front that eventually leads to initiation of a sprite streamer. Figure 1a shows the initial electron density distribution to model a sharp halo front between 70- and 75-km altitude with n 0 =2 × 10 7 m −3 , z 0 =73 km and σ z =300 m. At t =0, a constant electric field, E 0 =0.6 E k , simulating the the lightning and halo input is applied at 70-km altitude to start the simulation. As shown by Fig. 1b , the planar wave front is slightly shifted downwards and also sharpened at t =5 ms (see Supplementary Fig. 1 for the results at other moments of time). Figure 1: Sprite streamer initiation from a halo front deformed by mesospheric structures. ( a ) Initial electron density distribution. ( b ) A descending, sharpening halo front that keeps its planar geometry if there is no perturbation. ( c – h ) A growing mesospheric structure near the halo front that eventually leads to initiation of a sprite streamer. Full size image Streamer initiation from mesospheric structures As mentioned previously, neutral density fluctuations affect the dynamics of the electrical discharges by modifying the rate constants of the basic discharge processes. Here the effects of the mesospheric structures are taken into account by modifying electron impact ionization frequency in a horizontal atmospheric layer containing the halo front during a short or entire simulation period of time. The ionization frequency is multiplied by [1+ A cos( kr )], where A and k are the amplitude and wavenumber of the perturbed ionization frequency due to the mesospheric structures. Figure 1c–h shows that a streamer is initiated when a perturbation is introduced in a horizontal layer between 72- and 73-km altitude from 0 to 5 ms with A =0.5 and k =2 π /(2 km). As discussed previously, the values of both A and k are reasonable for the small-scale mesospheric structures generated by gravity waves. In Fig. 1c , a protrusion is developed from the wave front at the end of introduction of the perturbation. Figure 1d shows that the electric field is slightly enhanced around the tip of the perturbation. Now even if the modification of the ionization frequency is turned off, the perturbation continues to grow in terms of the magnitudes of the electron density and electric field. Figure 1e,f shows that at t =9.3 ms the electron density and electric field have significantly increased at the tip of the perturbation. The streamer is then initiated, and quickly propagates to the bottom boundary in 0.4 ms, as shown in Fig. 1g,h . This simulation is a theoretically simplified case to study the strength of the perturbation required to initiate streamers. Simulations with different magnitudes of the perturbation, applied fields, depths of the perturbed layer and durations of introducing the perturbation are presented below as well as in Supplementary Figs 2 and 3 . Although the detailed dynamics of the initiation process may be different (for example, the delay before the streamer initiation), the principal results are the same: sprite streamers can be initiated from small-scale ( ∼ 1–15 km) mesospheric structures produced by gravity waves near a halo front. It should be mentioned that although the simulation results presented here may appear to be similar to previous modelling studies on streamer initiation [14] , [18] , there are important differences. First, our work demonstrates that inhomogeneities are required and more importantly that small-scale neutral density perturbations created by gravity waves can initiate sprite streamers. Second, the electron detachment from O − ions [41] , [42] , [43] is included in our model. Without this process, it is impossible for a halo front to descend to 70- to 75-km altitude [41] , and furthermore, the perturbations are unable to grow to initiate streamers in the measurement-inferred lightning fields ( Supplementary Fig. 4 ). Therefore, the initiation of the long-delayed sprites near 70-km altitude could not be explained. 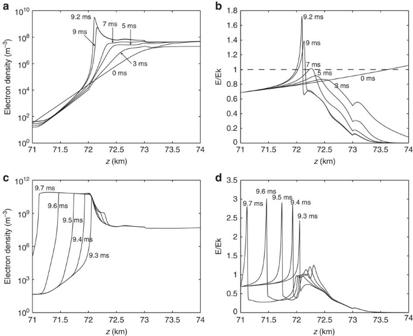Figure 2: Electron density and normalized electric field profiles on the symmetry axis. Parts (a) and (b) show the amplification of the perturbation before streamer initiation. Parts (c) and (d) show the initiation and propagation of a sprite streamer with standard features such as constant channel density and constant head field of about 3Ek. Figure 2 shows the electron density and normalized electric field profiles along the symmetry axis for the streamer initiation presented in Fig. 1 . Figure 2a,b illustrates the growth of the perturbation before streamer formation. The peak electron density and normalized electric field increase gradually, and the locations of the peaks also move slowly to lower altitude. The initial electric field is smaller than E k (that is, below the dashed line) everywhere except in a small region near 74-km altitude. It then becomes smaller than E k everywhere shortly after the simulation started, because the electric field quickly decreases in the high conductivity region near 74-km altitude. However, as shown by the field profiles at 3–5 ms, the peak electric field increases again because of the presence of the perturbation. Even after the modification of the ionization frequency is turned off at 5 ms, the peak field continues to increase and exceeds E k at 7 ms. Without the perturbation, the electric field would just decrease everywhere ( Supplementary Fig. 1 ) and streamer initiation would be impossible. A sharp field pulse is formed at 9.2 ms with a peak magnitude of about 1.7 E k , indicating that a streamer is forming. Figure 2c,d shows that at 9.3–9.4 ms the peak field reaches 2.5–3 E k and a positive streamer is fully formed. The streamer propagates to lower altitudes with an increasing speed and reaches the bottom boundary of the simulation domain in 0.3 ms. The average speed is 3 × 10 6 m s −1 , and the streamer channel density is about 8 × 10 10 m −3 . The head field, channel density, speed and acceleration of the streamer are consistent with previous streamer modelling results [10] , [15] , [16] , [21] , [22] , [25] . Figure 2: Electron density and normalized electric field profiles on the symmetry axis. Parts ( a ) and ( b ) show the amplification of the perturbation before streamer initiation. Parts ( c ) and ( d ) show the initiation and propagation of a sprite streamer with standard features such as constant channel density and constant head field of about 3 E k . Full size image Optical signatures of the streamer initiation The mean energy of the discharge electrons, which is a function of the local electric field, is about 2–3 eV near the initiation point of the streamer and 8 eV at the streamer head. Electrons with such energies can effectively excite air molecules through collisions, and photons are emitted when the excited air molecules fall back to their lower energy states, producing the light of sprites. The light of sprites is dominated by a spontaneous transition between two excited electronic states of N 2 molecules, known as the first positive band system of N 2 (1PN 2 ). The excitation threshold energy of the corresponding upper energy states is about 7.35 eV. As a result, strong optical emissions are produced both near the streamer initiation point and at the streamer head, where the electric field is large, as indicated by Fig. 3 showing the optical emission intensity distributions of 1PN 2 calculated from our simulation. The intensity is represented in Rayleighs that are the integrated photon emission rates along a line of sight, assumed to be horizontal here. A weak glow precedes the streamer initiation, and it descends downwards and shrinks a little as time progresses. After the initiation, as the streamer moves downwards, the brightness of both the streamer head and the initiation point increases. The figure shows that the maximal intensities of the streamer head and the preceding glow are on the order of 10 8 –10 9 R and 10 5 R, respectively. Given that the high-speed images are typically saturated at several tens of megaRayleighs with a dynamic range of 1,000 (refs 12 , 13 , 29 , 30 ), the streamer head would appear bright in high-speed images, while the preceding glow would hardly be visible. This conclusion is also consistent with the result from a recent analysis of high-speed images obtained with one of the most sensitive cameras currently in use in sprite observation. For streamers emerging out of a dark background, the analysis has indicated that the first detected streamer heads likely have already propagated a few kilometres [29] . Because the brightness of streamers exponentially increases, the streamer head at this time will be many times (a few tens) brighter than when it is just formed [16] , [22] . Therefore, the preceding glow and initial streamer head shown in Fig. 3 will not be detected by the current camera systems. 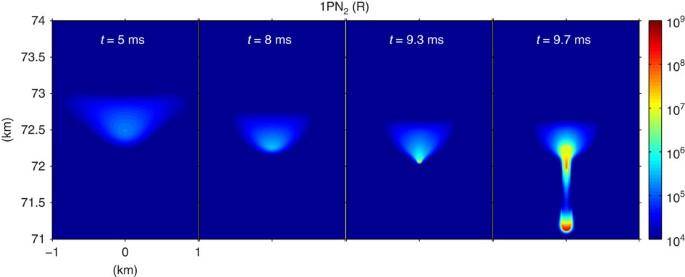Figure 3: 1PN2emission intensity associated with the streamer initiation. The diffuse glow preceding the streamer initiation is not bright enough to be detected by the current high-speed camera, and the streamer will appear to originate out of the dark background. Figure 3: 1PN 2 emission intensity associated with the streamer initiation. The diffuse glow preceding the streamer initiation is not bright enough to be detected by the current high-speed camera, and the streamer will appear to originate out of the dark background. Full size image Larger-scale mesospheric structures The kilometres-scale mesospheric structure considered above may correspond to the turbulent structures produced by gravity waves via breaking or instabilities. However, larger mesospheric perturbations such as the 5–15 km ‘ripple’ structures, resulting from the instability of gravity waves, can also initiate streamers. 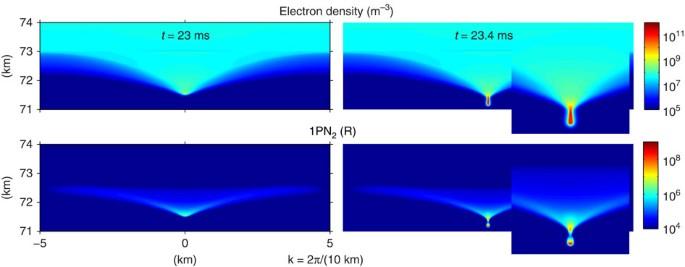Figure 4: Streamer initiation from perturbations with 10-km wavelength. The simulation is initialized withE0=0.6Ek,A=0.5 andk=2π/(10 km). The streamer initiation delays about 14 ms more than the previous streamer initiation case. Figure 4 shows initiation of a streamer from structures with a 10-km wavelength. The initializing parameters except the wavelength have the same values as those for the previous simulation case. The streamer initiation delays by about 23 ms or 14 ms more than the previous streamer initiation, suggesting that the growth rate for the smaller scale perturbation of the previous case is larger than the current case. Combined with the simulation results on planar wave propagation presented in Supplementary Fig. 1 , it can be expected that there exists a threshold for the perturbation scale length above which no streamers will be able to form. 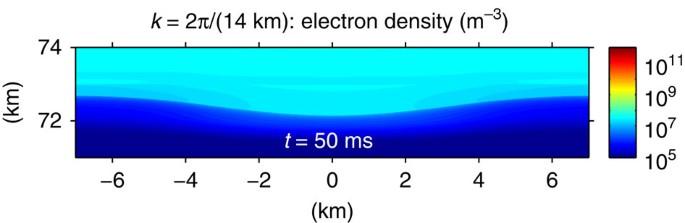Figure 5: No streamer initiation from perturbations with 14-km wavelength. The simulation is initialized withE0=0.6Ek,A=0.5 andk=2π/(14 km). Figure 5 shows that no streamer initiation occurs, if the wavelength is further increased to 14 km. Figure 4: Streamer initiation from perturbations with 10-km wavelength. The simulation is initialized with E 0 =0.6 E k , A =0.5 and k =2 π /(10 km). The streamer initiation delays about 14 ms more than the previous streamer initiation case. Full size image Figure 5: No streamer initiation from perturbations with 14-km wavelength. The simulation is initialized with E 0 =0.6 E k , A =0.5 and k =2 π /(14 km). Full size image Streamer initiation with a longer-lasting and deeper-perturbed layer Gravity waves at sprite initiation altitudes typically affect an atmospheric layer deeper than a few kilometres for a longer period of time [36] , [38] . 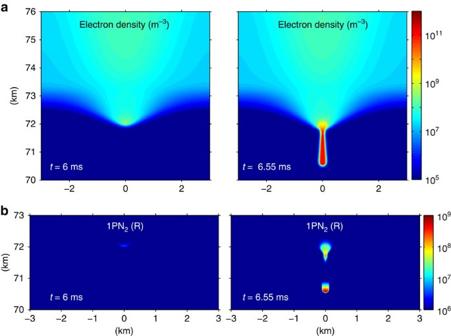Figure 6: Sprite streamer initiation from more realistic mesospheric perturbations. (a) Electron density distributions and (b) 1PN2emission intensity distributions. The perturbation in the ionization frequency is imposed throughout the simulation region and simulation period, andk=2π/(6 km). Figure 6 shows that the increases in the depth and lifetime of the perturbation layer do not change the principal results and conclusions of the paper. The simulation results are obtained with the same initializing parameters as those presented in Fig. 1 except that the simulation region is slightly larger, the perturbation in the ionization frequency is imposed throughout the simulation region and simulation period, and k =2 π /(6 km). In addition, the electric field at the bottom boundary of the simulation domain is gradually increased to −0.6 E k in 1 ms to more accurately model the condition imposed by the halo dynamics (see Methods). Compared with the results shown by Fig. 1 , the streamer initiation occurs about 3 ms earlier. The key for perturbing a halo front to initiate streamers is that the perturbation layer should be imposed near the front. If the perturbation layer is above or below the halo front, streamers will not be initiated. For example, additional simulation with imposing of the perturbation between 74 and 76 km altitude shows no streamer initiation. Note that the optical emission intensity is shown on a smaller intensity range than previous figures in order to clearly show that the current camera systems are not able to detect the weak glow before the streamer initiation of the long-delayed sprites. In addition, only the bottom half simulation region is shown for the optical emissions, because there are no visible emissions above. The intensity of the glow at 6 ms before streamer initiation is much weaker than the streamer head at 6.55 ms that has propagated more than 1 km distance, which is likely to be the first streamer head detected by intensified, high-speed cameras [29] . The intensity of the preceding glow is therefore below the detection limit of the current sprite observation systems, and this streamer will appear to emerge from a dark background. Figure 6: Sprite streamer initiation from more realistic mesospheric perturbations. ( a ) Electron density distributions and ( b ) 1PN 2 emission intensity distributions. The perturbation in the ionization frequency is imposed throughout the simulation region and simulation period, and k =2 π /(6 km). Full size image A long-delayed sprite preceded by a long-lasting halo The theory proposed here implies that some cases of the observed long-delayed sprites are preceded by a relatively stationary, long-lasting halo around 70-km altitude. Below, we present a unique observation of such an event. The event was recorded on 6 July 2011, from a close range of about 250 km, by two intensified high-speed cameras (see refs 29 , 30 for the details of the cameras) on two separate aircraft that flew at about 14-km altitude. The close range observation from an altitude above the lower dense atmosphere provided an optimal viewing condition to record dimmer structures. The simultaneous recordings with two high-speed cameras also allow accurate triangulation of the altitudes of the halo and the streamer. As shown by Fig. 7 , a streamer is initiated at about 70-km altitude from the bottom of a long-lasting halo that appears within 2–4 ms of the causative lightning and lasts about 10 ms. Note that, although appearing relatively bright in the intensity-clipped images of Fig. 7a,d , the halo is invisible when the original images are displayed on the full dynamic range of the pixel value. The initial streamer head is discernible in the original image as shown in Fig. 7c , whereas it saturates the clipped images in Fig. 7d . However, the main body of the sprite is so bright that even the original image is saturated. Overall, this observation shows that the intensities of halos, streamer heads and sprites vary over a very large range, and current high-speed camera systems cannot resolve them. However, it should be mentioned that their intensities also vary significantly between events [29] . 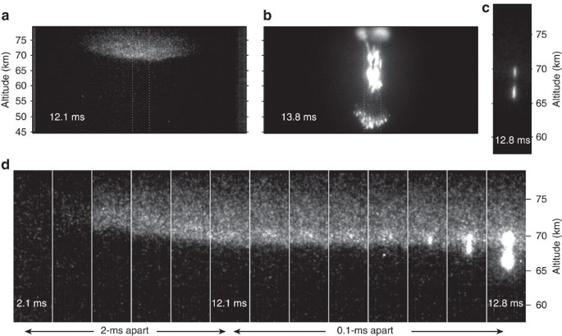Figure 7: A sprite preceded by a long-lasting halo observed on 6 July 2011. The times indicate the delay from the causative lightning. (a) A full field of view of the halo that appears within 2–4 ms of lightning and lasts about 10 ms. (b) The fully-developed sprite. (c) Streamer initiation at about 12 ms. (d) A successive sequence of images showing the halo and streamer initiation. Each image incanddcorresponds to the vertical strip bounded by the two dashes lines inaandb. Partsbandcshow the original images recorded with a dynamic change of 14 bits; and partsaanddshow the images processed by clipping the intensity values above 1,023 (that is, 10 bits). Figure 7: A sprite preceded by a long-lasting halo observed on 6 July 2011. The times indicate the delay from the causative lightning. ( a ) A full field of view of the halo that appears within 2–4 ms of lightning and lasts about 10 ms. ( b ) The fully-developed sprite. ( c ) Streamer initiation at about 12 ms. ( d ) A successive sequence of images showing the halo and streamer initiation. Each image in c and d corresponds to the vertical strip bounded by the two dashes lines in a and b . Parts b and c show the original images recorded with a dynamic change of 14 bits; and parts a and d show the images processed by clipping the intensity values above 1,023 (that is, 10 bits). Full size image Prompt sprite initiation The proposed theory can also be applied to initiation of prompt sprite streamers at higher altitudes. Because the streamers of prompt sprites are initiated during the rapidly descending stage of the halo, the initial density and field conditions previously used to model an almost stationary halo front are invalid. The measurement-confirmed night-time ionospheric density profile can be used to describe the ambient density condition before the causative lightning [44] , [45] . The profile is given by specifying an effective height of the lower ionosphere h ′ and the sharpness factor β (see Methods). In addition, it is also more accurate to use a time-varying E 0 ( t ) for the normal field component at the bottom boundary of the simulation domain. For example, E 0 ( t ) increases from 0 to its final value E 0 in a timescale of τ f (see Methods). 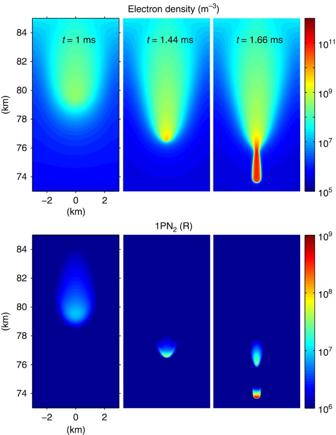Figure 8: Streamer initiation for prompt sprites. The perturbation in the ionization frequency is imposed throughout the simulation region and simulation period withA=1 andk=2π/(6 km). Figure 8 shows the simulation results of prompt streamer initiation. The simulation is initialized with A =1, k =2 π /(6 km), τ f =1 ms and E 0 =0.5 E k at 73 km altitude. The perturbation in the ionization frequency is imposed throughout the simulation region and simulation period. Note that the perturbation with A =0.5 leading to streamer initiation in previous cases does not initiate a streamer for the current simulation. In general, stronger perturbations are required to initiate streamers for a more smoothly varying initial density profile. The streamer forms slightly above 76-km altitude within 2 ms from applying the field. The glow before its initiation is brighter than the previous case, as shown in Fig. 3 , and it might be visible with the current camera system. It appears very similar to the luminous structures that lead to streamer initiation for prompt sprites. It can be expected that if the initial density profile is steeper, streamer initiation at higher altitude will be possible even with a weaker perturbation. The brightness of the preceding glow may also be increased by varying the values of k , β , E 0 and τ f . Overall, naturally existing, small-scale mesospheric structures can also lead to streamer initiation immediately following the causative lightning. Additional simulations to investigate various aspects of the initiation and the effects of the mesospheric structure properties are left for future studies. Figure 8: Streamer initiation for prompt sprites. The perturbation in the ionization frequency is imposed throughout the simulation region and simulation period with A =1 and k =2 π /(6 km). Full size image Our study indicates that sprite streamers can be initiated near a halo front from small-scale mesospheric neutral density perturbations of a few per cent change from the ambient value, such as those created by gravity waves. It should be noted that previous studies have also shown that, if strong, localized plasma perturbations with a density that is orders of magnitude higher than ambient electron density exist in the lower ionosphere, streamers can also be initiated from locations away from the halo front [20] , [21] , [22] , [23] , [25] , [26] . However, such ionization perturbations are unlikely to be present at initiation altitudes of the long-delay sprites. Our theory also naturally explains variable delay of sprite initiation, optical signatures of streamer initiation, and initiation of multiple isolated streamers from different locations. It also suggests that the optical signatures of sprite streamers emerging out of a dark background are not resolved by the current cameras used for sprite observation. Finally, although we only focus on studying streamer initiation from the mesospheric structures created by gravity waves, it can be expected that similar mesospheric structures generated by other atmospheric processes can also initiate sprite streamers. Since it is nearly impossible to observe the mesospheric structures at sprite initiation altitudes by other methods [36] , [38] , observational, theoretical and numerical studies of sprite streamer initiation can play an important role in investigating the properties of those structures. Plasma discharge model A cylindrically symmetric plasma discharge model is used to conduct the simulations presented. In this model, the dynamics of electrical discharges in the upper atmosphere are described by drift-diffusion equations of electrons and ions, coupled with Poisson’s equation[10]: where n e , n p and n n are electron, positive-ion and negative-ion number densities; v e =− μ e E is the drift velocity of electrons, with μ e being the absolute value of electron mobility and E being the electric field; D e is the electron diffusion coefficient; ν i is the ionization coefficient, ν a2 , and ν a3 are the two-body, and three-body attachment coefficients, respectively; β ep and β np are the coefficients of electron-positive ion and negative-positive ion recombinations, respectively; ν d is the frequency of electron detachment from O − ions [41] , [46] ; S ph is the electron-ion pair production rate due to photoionization; φ is the electric potential, e is the absolute value of electron charge and ɛ 0 is the permittivity of free space. Ions are assumed to be immobile for the timescales considered here because of their small mobilities. The coefficients of the model are assumed to be a function of the local electric field and are obtained from the solution of the Boltzmann equation [47] . The numerical methods used to solve the model equations were described previously [10] except that for calculating S ph (refs 48 , 49 ). Note that the electron detachment from O − ions was found to be important only recently [41] , [42] , [43] , and it was not included in early modelling work of electrical discharges at high altitudes. Boundary conditions To imitate the physical conditions imposed by the lightning and the halo on sprite streamer initiation, the following boundary conditions are implemented for Poisson’s equation: The simulation domain corresponds to a small cylinder at the bottom of a descending halo front. The top boundary is located behind the halo front, where electron density is large, and is approximated by a perfectly conducting surface with φ =0 V. The bottom boundary is below the halo front, where electron density is small, and the electric field, dominated by the vertical component, changes very slowly over time [41] . Therefore, the vertical field component at the bottom boundary is set to be a constant value scaled from − E 0 at 70-km altitude, where N 70 and N bottom are the air neutral densities at 70-km altitude and the bottom boundary, respectively. The value of E 0 can be varied depending on the strength of the parent CG lightning. The halo simulation reported previously [41] gives E 0 ≃ 0.5–0.6 E k . The outer boundary condition states that the horizontal components of the electric field are zero, which is appropriate for modelling planar wave front propagation. Initial conditions The initial density profiles of electrons and ions to model a halo front at an intermediate stage of propagation are described with a hyperbolic tangent profile: Typical values of the parameters used in our simulations are n 0 =2 × 10 7 m −3 , z 0 =73 km and σ z =300 m. Implementation of mesospheric structures The effects of the mesospheric structures such as those produced by gravity waves are taken into account by modifying the electron impact ionization frequency in a horizontal layer ( z 1 < z < z 2 ) containing the halo front in a prescribed simulation period as follows: where ν i0 is the ionization frequency calculated directly with the electric field. By modifying the ionization frequency to introduce mesospheric structures in the simulation, it is guaranteed that equal numbers of electrons and positive ions are added, avoiding introducing a net amount of charge to the system. It should be noted that, under the cylindrical symmetry assumption of our model, the perturbation imposed this way consists of concentric rings. A fully 3D model is needed to model arbitrary perturbations. Initial and boundary conditions for simulating prompt streamer initiation A standard, ambient ionospheric density profile is used to represent the condition before the causative lightning: where n 0 =1.43 × 10 13 m −3 , h ′=85 km, and β =0.5 km −1 . The normal component of the electric field at the bottom boundary of the simulation domain is gradually increased to its final value E 0 by using the following formula, which is commonly employed to describe the driving source for modelling sprites or halos: where E 0 is the final value of E 0 ( t ) and τ f is the timescale for E 0 ( t ) to reach E 0 . How to cite this article : Liu, N. et al. Sprite Streamer Initiation from Natural Mesospheric Structures. Nat. Commun. 6:7540 doi: 10.1038/ncomms8540 (2015).